Metal-centred azaphosphatriptycene gear with a photo- and thermally driven mechanical switching function based on coordination isomerism Metal ions can serve as a centre of molecular motions due to their coordination geometry, reversible bonding nature and external stimuli responsiveness. Such essential features of metal ions have been utilized for metal-mediated molecular machines with the ability to motion switch via metallation/demetallation or coordination number variation at the metal centre; however, motion switching based on the change in coordination geometry remain largely unexplored. Herein, we report a Pt II -centred molecular gear that demonstrates control of rotor engagement and disengagement based on photo- and thermally driven cis – trans isomerization at the Pt II centre. This molecular rotary motion transmitter has been constructed from two coordinating azaphosphatriptycene rotators and one Pt II ion as a stator. Isomerization between an engaged cis -form and a disengaged trans -form is reversibly driven by ultraviolet irradiation and heating. Such a photo- and thermally triggered motional interconversion between engaged/disengaged states on a metal ion would provide a selector switch for more complex interlocking systems. Transmission of rotary motion is a key process of molecular machines [1] , [2] , [3] . To correlate two or more movable elements in a controllable manner, a stator, which can bring them appropriately close to each other, is a key part of motion. A significant number of excellent examples have been reported on synthetic molecular gearing systems with intramolecularly correlated rotators [4] , [5] , [6] , [7] , [8] , [9] . However, the control of rotary transmission between molecular rotators is still in an early phase [10] , [11] , and therefore, in particular, switchable motion transmission is a challenge. Dynamic engagement between rotators is a typical rotary transmission in molecular machines. Triptycene is a well-known part of gear molecules with a rigid, highly symmetrical paddlewheel structure. More than one triptycene rotators can be covalently connected with an organic stator designed so as to have a proper positional relationship between the connected rotators [12] , [13] , [14] , [15] , [16] , [17] , [18] , [19] , [20] , [21] . Another unique example of covalently linked systems is a silicon-centred bistriptycene system [19] , which undergoes switchable gearing triggered by a chemical stimulus, fluorination/defluorination. We focused on metal ions as a control element of molecular motions due to their essential features such as reversible bonding natures with ligands, dynamic ligand exchange and external stimuli responsiveness [22] , [23] , [24] . A certain number of excellent examples of metal-mediated molecular machines capable of motion switching via metallation/demetallation or coordination number variation on the metal centre have been reported [25] , [26] , [27] . Herein, we report a Pt II -centred molecular gear that demonstrates control of rotor engagement and disengagement based on photo- and thermally driven cis – trans isomerization at the Pt II centre. This molecular rotary motion transmitter has been constructed from two coordinating azaphosphatriptycene rotators and one Pt II ion as a stator. Isomerization between an engaged cis -form and a disengaged trans -form is reversibly driven by ultraviolet irradiation and heating. Such a photo- and thermally triggered motional interconversion between engaged/disengaged states on a metal ion would provide a selector switch for more complex interlocking systems. Design of metal-centred molecular gear In this study, we have developed a metal-centred molecular gear PtCl 2 1 2 , in which two ligands as rotators, 2-methoxy-9-aza-10-phosphatriptycene ( 1 ), directly bind to the Pt II stator [28] , [29] . One striking feature of this system is a clutch-like function that allows switching of the engagement of the two rotators based on photo- and thermally driven cis – trans isomerization on the Pt II centre in a traceless manner with no chemical by-products ( Fig. 1 ) [30] , [31] . 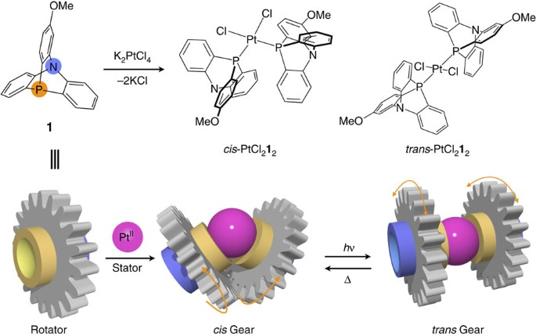Figure 1: Schematic representation of a PtII-centred molecular gear PtCl212. This molecular gear has two azaphosphatriptycene rotators coordinating to the central PtIIion as a stator. Isomerization between an engagedcis-form and a disengagedtrans-form are reversibly driven by ultraviolet irradiation at 360 nm and heating. Figure 1: Schematic representation of a Pt II -centred molecular gear PtCl 2 1 2 . This molecular gear has two azaphosphatriptycene rotators coordinating to the central Pt II ion as a stator. Isomerization between an engaged cis -form and a disengaged trans -form are reversibly driven by ultraviolet irradiation at 360 nm and heating. Full size image Synthesis of azaphosphatriptycene ligand 2-Methoxy-9-aza-10-phosphatriptycene ( 1 ), in which the bridgehead positions of triptycene are replaced by a nitrogen and a phosphorus atoms, was chosen as a ligand-type rotator [32] . The rotator 1 was synthesized from 3-anisidine in four steps in 9% overall yield, and was characterized by 1 H, 13 C and 31 P nuclear magnetic resonance (NMR) spectroscopy, electrospray ionization-mass spectrometry and elemental analysis ( Supplementary Figs 1–10 ). We expected that when two rotators 1 as monodentate phosphine ligands bind to a compatible Pt II ion in a cis position, they should gear with each other. Preparation and characterization of Pt II complexes The reaction of rotator 1 and 0.5 eq of K 2 PtCl 4 in EtOH/H 2 O (1/1, v v −1 ) at room temperature for 21 h afforded a mixture of square-planar Pt II –phosphine complexes, cis -PtCl 2 1 2 and a small amount of trans -PtCl 2 1 2 ( Figs 1 , 2a ). After recrystallization from CHCl 3 /diethyl ether, pure cis -PtCl 2 1 2 was successfully obtained as colourless crystals in 59% yield ( Supplementary Figs 11 and 13 ). The coordinating donor atom and the geometry around the Pt II centre in solution were determined by NMR spectroscopy. In a 31 P NMR spectrum of the cis isomer in C 6 D 6 , a 31 P- 195 Pt coupling was observed ( J 1 =3,625 Hz; Supplementary Fig. 12 ) due to the binding of phosphine ligand to the central Pt II ion. Then, a 1 H NMR spectrum of the cis isomer showed that the proton signals for the 3-positions of azaphosphatriptycene shifted upfield from the free ligand, indicating that two azaphosphatriptycene ligands were close to each other. Moreover, a lineshape analysis of the spectral pattern of the proton signals of the 4-positions suggests that there are two rotational isomers, meso and dl forms, in a 1:2 ratio in solution ( Fig. 2b , Supplementary Fig. 14 ). We analysed the kinetics of the gear slippage during interconversion between meso and dl isomers of cis -PtCl 2 1 2 . Variable temperature 1 H NMR measurement of cis -PtCl 2 1 2 was described by the two-signal overlap model of the meso and dl isomers. An Eyring plot of the exchange rates of the isomers at every temperature gave activation parameters of the interconversion, Δ H ‡ =16.4±0.2 kcal·mol −1 and Δ S ‡ =−0.9±0.7 cal·K −1 ( Fig. 2c , Supplementary Fig. 15 ). The enthalpy value is significantly lower than the reported value for covalently connected triptycene gears [15] , [19] . 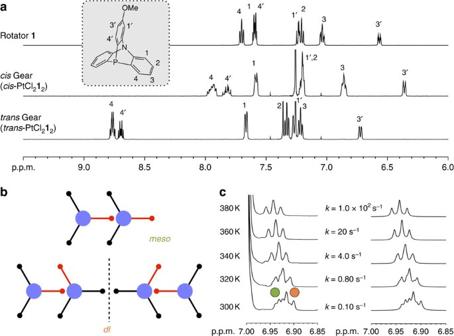Figure 2:1H NMR spectra of rotator 1 andcis- andtrans-PtCl212. The signals of a methoxy group of rotator1(∼3.8 p.p.m.) are omitted for clarity. For the whole NMR spectra, see theSupplementary Figures 7, 11 and 16. (a)1H NMR spectrum of (i)1, (ii)cis-PtCl212and (iii)trans-PtCl212(500 MHz, CDCl3, 300 K). The1H NMR spectra ofcis-PtCl212includemesoanddlisomers in a∼1:2 ratio. (b) Isomerism based on rotational conformation. (c) Observed and simulated spectra of 3-positions' proton at varied temperatures (500 MHz, TCE-d2/toluene-d8=1:1). Left: observed spectra in the range from 380 to 300 K. Right: simulated spectra based on the two-state exchange model. Green and orange circles denotemesoanddlisomers, respectively. Figure 2: 1 H NMR spectra of rotator 1 and cis - and trans -PtCl 2 1 2 . The signals of a methoxy group of rotator 1 ( ∼ 3.8 p.p.m.) are omitted for clarity. For the whole NMR spectra, see the Supplementary Figures 7, 11 and 16 . ( a ) 1 H NMR spectrum of (i) 1 , (ii) cis -PtCl 2 1 2 and (iii) trans -PtCl 2 1 2 (500 MHz, CDCl 3 , 300 K). The 1 H NMR spectra of cis -PtCl 2 1 2 include meso and dl isomers in a ∼ 1:2 ratio. ( b ) Isomerism based on rotational conformation. ( c ) Observed and simulated spectra of 3-positions' proton at varied temperatures (500 MHz, TCE- d 2 /toluene- d 8 =1:1). Left: observed spectra in the range from 380 to 300 K. Right: simulated spectra based on the two-state exchange model. Green and orange circles denote meso and dl isomers, respectively. Full size image It is noteworthy in connection with motion transmission that a certain number of Pt II complexes display photo-driven cis / trans isomerization [30] , [31] . Under photoirradiation at 360 nm, cis -PtCl 2 1 2 was found to be isomerized to trans -PtCl 2 1 2 in C 6 H 6 at room temperature ( cis / trans =50:50 by 1 H NMR in CDCl 3 at 300 K). As a result of slow evaporation, trans -PtCl 2 1 2 was isolated as yellow crystals in 29% yield ( Supplementary Figs 16 and 17 ). In a 31 P NMR spectrum of the trans isomer in CDCl 3 , a 31 P- 195 Pt coupling ( J 1 =2,937 Hz, in Supplementary Fig. 18 ) indicated that the two phosphine ligands bind to the central Pt II ion. On the other hand, its 1 H NMR spectrum in CDCl 3 showed neither splitting nor upfield shift of the proton signals for the 4-positions, suggesting the absence of significant intramolecular interactions between the two rotators. X-ray crystallographic analyses Crystals of cis -PtCl 2 1 2 ·(ether) suitable for single-crystal X-ray structure analysis were obtained by liquid–liquid diffusion of Et 2 O into a solution of PtCl 2 1 2 in toluene. One molecule of diethyl ether was included into the unit structure ( Fig. 3 , Supplementary Fig. 19 ). The X-ray diffraction data demonstrated that the two rotators adopt an ‘engaged’ cis form in the solid state. A unit cell consists of a meso isomer of PtCl 2 1 2 , one rotational isomer comes from tight meshing of the two rotators. Notably, intramolecular CH–π interactions were observed between the two rotators. Each Pt II ion is in a distorted square planar geometry, in which the P–Pt–P angle is over 90° (99.95(5)°) due to the bulkiness of rotator 1 . The two rotators 1 are thus suitably engaged with each other on the Pt II stator. In contrast, single-crystal X-ray structure analysis of trans -PtCl 2 1 2 ·(C 6 H 6 ) 2 revealed that the two phosphine ligands as rotators are across from one another in the square planar Pt II complex ( Supplementary Fig. 20 ). This photoisomerized trans form can be regarded as a ‘disengaged’ state of the metal-centred molecular gear. 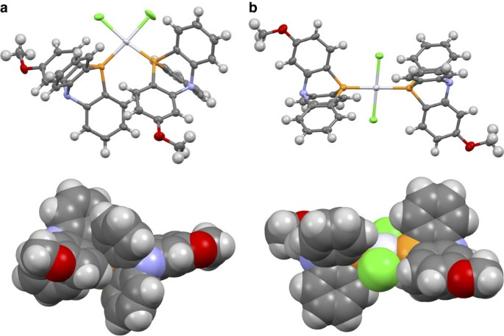Figure 3: X-ray crystal structures ofcis- andtrans-PtCl212. (a)cis-PtCl212·(ether). (b)trans-PtCl212·(C6H6)2. In both cases, the structures are indicated as ORTEP (Oak Ridge Thermal Ellipsoid Plot) diagram with 50% thermal ellipsoid (upper) and space-filling model (bottom). Solvents are omitted for clarity, and colours are coded according to CPK (Corey, Pauling, Koltun) colouring. Figure 3: X-ray crystal structures of cis - and trans -PtCl 2 1 2 . ( a ) cis -PtCl 2 1 2 ·(ether). ( b ) trans -PtCl 2 1 2 ·(C 6 H 6 ) 2 . In both cases, the structures are indicated as ORTEP (Oak Ridge Thermal Ellipsoid Plot) diagram with 50% thermal ellipsoid (upper) and space-filling model (bottom). Solvents are omitted for clarity, and colours are coded according to CPK (Corey, Pauling, Koltun) colouring. Full size image Photo- and thermally driven isomerization of PtCl 2 1 2 We then envisioned that this gear system could be applied to a stimuli-responsive molecular switch based on the photo- and thermally driven cis – trans isomerization in an appropriate solvent. It is well known that photo or thermal isomerization of diphosphine Pt II complexes highly depends on the solvent polarity [8] . Polar solvents generally prefer cis form rather than trans form because the cis complex has a dipole moment that interacts better with the solvent polarity. Photo-driven isomerization from cis to trans form was then examined in a solvent with low polarity. Ultraviolet light at 360 nm was irradiated to a solution of pure cis -PtCl 2 1 2 in toluene- d 8 at room temperature ( Fig. 4a,b ). A photo stationary state was reached after 30 min, where the cis / trans ratio was changed to 15:85 ( Supplementary Fig. 21 ). On the other hand, in more polar 1,1,2,2,-tetrachloroethane- d 2 (TCE- d 2 ), thermal isomerization from trans to cis was so fast in the dark at room temperature that it was difficult to obtain a 1 H NMR spectrum of pure trans complex in the TCE- d 2 solution because of the rapid isomerization to the cis form. After 10 h, the trans complex was transformed into cis form nearly quantitatively ( cis / trans =98:2; Supplementary Fig. 22 ). This structural interconversion was repeatable in a mixed solvent of TCE- d 2 /toluene- d 8 =1:1. When a solution of pure cis -PtCl 2 1 2 was irradiated by ultraviolet light at 360 nm, the cis to trans conversion proceeded smoothly at room temperature, and the reaction achieved its equilibrium ( cis / trans =19:81) in 30 min. In this mixed solvent system, the interconversion from trans to cis was slow enough to determine the ratio of the complex by NMR at 300 K. When the trans -based solution was heated at 100 °C for 10 h, the trans -based solution was reversed to the cis -based solution with the cis / trans =78:22. This cis – trans isomerization process was thus repeatable at least three times by the repetition of stimuli ( Fig. 4c and Supplementary Figs 23 and 24 ). 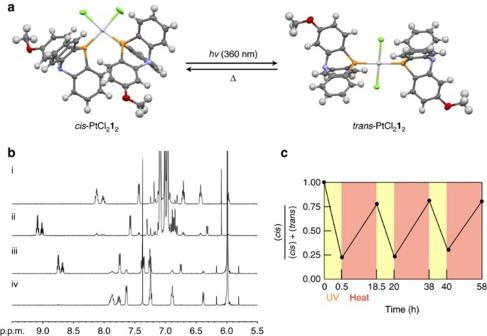Figure 4: Photo and thermal switching of molecular gear PtCl212. (a) Photo- and thermally induced isomerization betweencis- andtrans-PtCl212. (b)1H NMR spectra for photo- and thermally induced isomerization fromcis- totrans-PtCl212(500 MHz, 300 K). (i) A solution of single crystals ofcis-PtCl212in toluene-d8(cis/trans=99:1); (ii) a solution of (i) after photoirradiation at 360 nm (after 30 min,cis/trans=15:85); (iii) a solution of single crystals oftrans-PtCl212in TCE-d2(after 5 min,cis/trans=12:88); (iv) a solution of (iii) after 10 h at room temperature (cis/trans=2:98). (c) Reversible switching of the molecular gearing system, PtCl212, in TCE-d2/toluene-d8=1:1 (v v−1). Figure 4: Photo and thermal switching of molecular gear PtCl 2 1 2 . ( a ) Photo- and thermally induced isomerization between cis - and trans- PtCl 2 1 2 . ( b ) 1 H NMR spectra for photo- and thermally induced isomerization from cis - to trans- PtCl 2 1 2 (500 MHz, 300 K). (i) A solution of single crystals of cis -PtCl 2 1 2 in toluene- d 8 ( cis / trans =99:1); (ii) a solution of (i) after photoirradiation at 360 nm (after 30 min, cis / trans =15:85); (iii) a solution of single crystals of trans -PtCl 2 1 2 in TCE- d 2 (after 5 min, cis / trans =12:88); (iv) a solution of (iii) after 10 h at room temperature ( cis / trans =2:98). ( c ) Reversible switching of the molecular gearing system, PtCl 2 1 2 , in TCE- d 2 /toluene- d 8 =1:1 (v v −1 ). Full size image In conclusion, we have developed a molecular gear, PtCl 2 1 2 , composed of two azaphosphatriptycene rotators 1 with a Pt II ion acting as a stator. The repeatable mechanical switching function based on the cis – trans isomerization at the Pt II centre was achieved by photoirradiation and heating. Traceless external stimuli-responsive configurational changes of metal ions show promise as a movement element of molecular machines with a motion transmission function. General information Unless otherwise noted, solvents and reagents were purchased and used without further purification. 2-Methoxy-9-aza-10-phosphatriptycene ( 1 ) was synthesized from 3-anisidine ( Supplementary Figs 1–10 and Supplementary Note 1 ). 1 H, 13 C, 31 P NMR and other two-dimensional NMR spectra were recorded on a Bruker AVANCE III-500 (500 MHz) spectrometer. Tetramethylsilane was used as an internal standard ( δ 0 p.p.m.) for 1 H and 13 C NMR measurements when CDCl 3 was used as solvent. A residual solvent signal was used for calibration of 1 H NMR measurements when other deuterated solvents (C 6 HD 5 : 7.16 p.p.m. ; toluene- d 7 : 6.97 p.p.m. ; 1,1,2,2-tetrachloroethane- d : 5.99 p.p.m.) was used as a solvent. ESI-TOF mass data were recorded on a Micromass LCT Premier XE mass spectrometer. Unless otherwise noted, experimental conditions were as follows: ion mode, positive; capillary voltage, 3,000 V; sample cone voltage, 30 V; desolvation temperature, 150 °C; source temperature, 80 °C). Melting point was measured by Yanaco Micro Melting Point Apparatus MP-500D and uncorrected. Elemental analysis was conducted in the Microanalytical Laboratory, Department Chemistry, Graduate School of Science, the University of Tokyo (Tokyo, Japan). Infrared spectra were recorded on a Jasco FT/IR 4,200 with an ATR equipment. Synthesis of cis -PtCl 2 1 2 To a 5.0 mM solution of K 2 PtCl 4 /H 2 O (40 ml, 0.20 mmol, 1.0 eq) was added a 10 mM solution of 2-methoxy-9-aza-10-phosphatriptycene ( 1 ) in EtOH (40 ml, 0.40 mmol, 2.0 eq). The suspended solution was then stirred at room temperature for 21 h in the dark. The resulting precipitate was collected by filtration, washed with H 2 O and EtOH, and dried under vacuum to give a colourless solid (144 mg). The crude product was purified by recrystallization from chloroform/diethyl ether to give cis -PtCl 2 1 2 (112 mg, 0.118 mmol, 59%) as a colourless solid. 1 H NMR (C 6 D 6 , 500 MHz, 300 K): δ 7.81–7.78 (m, 4H), 7.71–7.66 (m, 2H), 7.05 (d, J =7.6 Hz, 4H), 6.83 (s, 2H), 6.31–6.27 (m, 4H), 6.04–6.00 (m, 4H), 5.62–5.68 (m, 2H), 2.57 (s, 2H), 2.55 (s, 4H); 31 P NMR (C 6 D 6 , 202 MHz, 300 K): δ −31.0 ( J P–Pt =3,625 Hz); HRMS (CHCl 3 /CH 3 CN/HCO 2 H, positive): [PtCl 1 2 ] + (C 38 H 28 ClN 2 O 2 P 2 Pt) m / z 836.0958 (required, 836.0957). Synthesis of trans -PtCl 2 1 2 In a 50 ml three-necked flask, a solution of cis -PtCl 2 1 2 (20.0 mg, 21 μmol) in benzene was irradiated at 360 nm for 1 h at room temperature. The solvent was removed by evaporation to give a yellow solid (22.5 mg). The crude product was recrystallized from benzene (2 ml) to obtain yellow crystals of trans -PtCl 2 1 2 ·(C 6 H 6 ) 2 . After dryness, 5.8 mg of desired complex was obtained, which contains 0.5 eq of benzene (confirmed by NMR, 6.1 μmol, 29%). 1 H NMR (CDCl 3 , 500 MHz, 300 K): δ 8.78–8.75 (m, 4H), 8.70 (dt, J =8.4, 5.4 Hz, 2H), 7.66 (dd, J =7.7, 1.1 Hz, 4H), 7.34 (td, J =7.6, 1.2 Hz, 4H), 7.28–7.25 (m, 2H), 7.22 (td, J =7.5, 1.3 Hz, 4H), 6.72 (dt, J =8.4, 1.2 Hz, 2H), 3.82 (s, 6H); 31 P NMR (CDCl 3 , 202 MHz, 300 K): δ −39.0 ( J P–Pt =2,937 Hz); HRMS (CHCl 3 /CH 3 CN/HCO 2 H, positive): [PtCl 1 2 ] + (C 38 H 28 ClN 2 O 2 P 2 Pt) m / z 836.0958 (required, 836.0957). Photo- and thermally driven isomerization of PtCl 2 1 2 A 1.0 mM solution of cis -PtCl 2 1 2 in TCE- d 2 /toluene- d 8 =1:1 (600 μl, 0.60 μmol) and a 100 mM solution of 1,4-dioxane in TCE- d 2 /toluene- d 8 =1:1 (6.0 μl, 0.60 μmol) were placed in an NMR tube, which was sealed by a septum rubber and degassed by freeze–pump–thaw three times. The reaction mixture was irradiated with ultraviolet lamp (ASAHI, MAX-303) using 360 nm filter (bandwidth=10 nm) at room temperature, and was heated at 100 °C in the dark ( Supplementary Figs 19–22 ). X-ray diffraction analysis Single-crystal X-ray crystallographic analyses were performed using a Rigaku Saturn724+ diffractometer with MoK α radiation (for cis -PtCl 2 1 2 ) or Rigaku RAXIS-RAPID imaging plate diffractometer with MoK α radiation (for trans -PtCl 2 l 2 ), and obtained data were calculated using the Crystal Structure crystallographic software package except for refinement, which was performed using SHELXL-2014 (ref. 33 ). All hydrogen atoms were placed geometrically and refined using a riding model. Details for the synthesis and X-ray diffraction mesurements of both cis - and trans -complex are given in CIF files and Supplementary Figs 19 and 20 and Supplementary Note 2 . Data availability Crystallographic data in this paper can be obtained free of charge from the Cambridge Crystallographic Data Centre ( http://www.ccdc.cam.ac.uk/data_request/cif ). The Deposit numbers are 1404948 ( cis -PtCl 2 1 2 ) and 1404949 ( trans -PtCl 2 1 2 ), respectively. All other data are available on this article and its Supplementary Information file. How to cite this article: Ube, H. et al . Metal-centred azaphosphatriptycene gear with a photo- and thermally driven mechanical switching function based on coordination isomerism. Nat. Commun. 8, 14296 doi: 10.1038/ncomms14296 (2017). Publisher’s note : Springer Nature remains neutral with regard to jurisdictional claims in published maps and institutional affiliations.